Regulation of adipose oestrogen output by mechanical stress Adipose stromal cells are the primary source of local oestrogens in adipose tissue, aberrant production of which promotes oestrogen receptor-positive breast cancer. Here we show that extracellular matrix compliance and cell contractility are two opposing determinants for oestrogen output of adipose stromal cells. Using synthetic extracellular matrix and elastomeric micropost arrays with tunable rigidity, we find that increasing matrix compliance induces transcription of aromatase, a rate-limiting enzyme in oestrogen biosynthesis. This mechanical cue is transduced sequentially by discoidin domain receptor 1, c-Jun N-terminal kinase 1, and phosphorylated JunB, which binds to and activates two breast cancer-associated aromatase promoters. In contrast, elevated cell contractility due to actin stress fibre formation dampens aromatase transcription. Mechanically stimulated stromal oestrogen production enhances oestrogen-dependent transcription in oestrogen receptor-positive tumour cells and promotes their growth. This novel mechanotransduction pathway underlies communications between extracellular matrix, stromal hormone output, and cancer cell growth within the same microenvironment. The mechanical phenotype of a cell is defined by cytoskeletal forces generated by the cell in response to physical cues from the extracellular matrix (ECM) [1] . During organogenesis, reciprocal interactions between intra- and extracellular forces regulate cell contractility, proliferation, differentiation and other cellular functions [2] . Accumulating evidence also suggests that altered mechanical phenotype is associated with development of different pathological conditions. For example, increased rigidity of tumour cells and their surrounding tissue microenvironment can enhance the migratory and invasive properties of tumour cells per se [3] , [4] , [5] . In contrast, how mechanical phenotype influences host stromal cells and their ensuing communication with tumour cells is poorly understood. Prolonged exposure to elevated local and circulating oestrogens is a well-recognized disease-promoting factor for breast cancer. Although the ovary is the major contributor of circulating oestrogens in pre-menopausal women, extraovarian oestrogens are overproduced in adipose stromal cells (ASCs) adjacent to breast tumours and in adipose tissue of cancer-free obese women [6] . In fact, excessive oestrogen production by adipose tissue is considered to be the primary contributing factor for obesity-associated breast cancer risk among postmenopausal women [6] . Aromatase catalyses the conversion of androgens to oestrogens, the last and rate-limiting step in oestrogen biosynthesis. Therefore, levels of local and circulating oestrogens are, to a large extent, dictated by aromatase abundance. Aromatase is normally expressed in selective cell and tissue types through the actions of several tissue-specific transcription promoters [6] , [7] , [8] . Aromatase inhibitors (AIs) are the most efficacious endocrine therapy for treating oestrogen receptor α-positive (ER+) breast cancer in postmenopausal women [9] , [10] , [11] , [12] , underscoring the clinical relevance of extraovarian aromatase overexpression. Tumour-secreted soluble factors are known to stimulate aromatase transcription in ASCs and enhance oestrogen biosynthesis [13] , [14] , [15] , [16] . In addition to these biochemical cues, altered mechanical phenotype occurs in extraovarian pathologies that are associated with aromatase overexpression, including breast cancer [5] , endometriosis [17] , [18] , [19] and uterine fibroids [20] , [21] , [22] . This raises the possibility that biomechanical signalling in the tissue microenvironment may serve as a distinct cue to stimulate aromatase transcription and oestrogen production. In the current study, we combine bioengineering and molecular tools to investigate the impact of mechanical phenotype on oestrogen output from ASCs and the functional consequences in terms of proliferation of ER+ breast tumour cells. Our work uncovers a previously unappreciated mechanotransduction mechanism that converts biomechanical signals to elevated endocrine/paracrine production in ASCs, which in turn stimulates the proliferation of ER+ breast tumour cells. ECM stimulates stromal oestrogen biosynthesis To investigate how mechanical phenotype affects adipose oestrogen biosynthesis, we isolated primary ASCs from human breast and abdominal fat tissue, and embedded them within type 1 collagen-based, three-dimensional (3-D) gels or on conventional plastic two-dimensional (2-D) cell culture plates. ASCs in a 3-D microenvironment expressed much higher levels of aromatase mRNA and protein ( Fig. 1a ) than their counterparts in the 2-D condition. When an aromatase substrate was included in the culture medium, cells in 3-D, but not 2-D, produced an appreciable amount of oestrogens ( Fig. 1c ). Importantly, the 3-D-induced oestrogen production was completely abrogated by an aromatase-specific inhibitor letrozole ( Fig. 1c ). Thus, the collagen-based 3-D system significantly enhances aromatase expression and stromal oestrogen output. 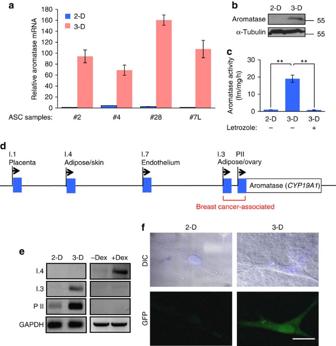Figure 1: ECM stimulates aromatase transcription and oestrogen biosynthesis in ASCs. (a) 3-D ASCs express much higher aromatase mRNA than 2-D cells. (b) Aromatase protein is induced in 3-D ASCs. (c) Aromatase enzymatic activity is significantly elevated in 3-D ASCs. (d) Illustration of the relevant tissue-specific promoters of the aromatase (CYP19A1) gene. (e) Determination of the promoter usage in ECM-activated aromatase transcription. Dexamethasone (Dex; 1 μM) treatment for 24 h is used as a positive control for I.4-specific transcripts. (f) ECM-induced GFP expression in ASCs integrated with the I.3/PII-GFP reporter. The blue colour in differential interference contrast (DIC) represents DAPI-stained nuclei. **P<0.01, Student’st-test. Data represent mean±s.e.m. of three independent experiments. Scale bar, 30 μm. Figure 1: ECM stimulates aromatase transcription and oestrogen biosynthesis in ASCs. ( a ) 3-D ASCs express much higher aromatase mRNA than 2-D cells. ( b ) Aromatase protein is induced in 3-D ASCs. ( c ) Aromatase enzymatic activity is significantly elevated in 3-D ASCs. ( d ) Illustration of the relevant tissue-specific promoters of the aromatase ( CYP19A1 ) gene. ( e ) Determination of the promoter usage in ECM-activated aromatase transcription. Dexamethasone (Dex; 1 μM) treatment for 24 h is used as a positive control for I.4-specific transcripts. ( f ) ECM-induced GFP expression in ASCs integrated with the I.3/PII-GFP reporter. The blue colour in differential interference contrast (DIC) represents DAPI-stained nuclei. ** P <0.01, Student’s t -test. Data represent mean±s.e.m. of three independent experiments. Scale bar, 30 μm. Full size image Tissue-selective expression of aromatase is controlled by a number of transcription promoters ( Fig. 1d ) [6] . For example, an adipose tissue-specific, glucocorticoid-inducible promoter (I.4) is responsible for relatively low levels of aromatase transcription in normal adipose tissue [6] . When exposed to tumour cell-secreted factors, two potent and closely positioned promoters (I.3 and PII) are aberrantly activated in ASCs, resulting in increased oestrogen biosynthesis [6] . We found that the 3-D microenvironment specifically induced the breast cancer-associated promoters I.3/PII ( Fig. 1e ). In contrast, the I.4 promoter was not stimulated at all by 3-D ECM, despite its robust response to dexamethasone (a synthetic analogue of glucocorticoid) ( Fig. 1e ). Furthermore, when the I.3/PII promoter fragment was fused with a green fluorescent protein (GFP) reporter and integrated into primary ASCs, GFP-positive cells were readily detected under the 3-D, but not 2-D condition ( Fig. 1f and Supplementary Fig. S1 ). These data suggest that the 3-D microenvironment recapitulates breast cancer-associated, promoter-specific activation of aromatase transcription. Matrix compliance is a stimulus of aromatase transcription Cells adopt a certain degree of contractility in response to topological (3-dimensionality), biochemical (ligand–receptor interaction), and biomechanical cues (rigidity/compliance) presented by ECM ( Fig. 2a ). We therefore sought to discern the contribution of each of these ECM-related parameters to aromatase transcription. To determine whether dimensionality influences stromal aromatase expression, we cultured ASCs in a ‘2.5-D’ gel [23] , [24] , where an additional layer of collagen was deposited on the apical side of collagen-overlaid ASCs ( Fig. 2b ). ASCs sandwiched within this 2.5-D system lacked true 3-dimensionality yet maintained comparable cell–matrix contact and matrix compliance as compared with those in 3-D gels. ASCs in these two topologically distinct systems expressed similar levels of aromatase mRNA ( Fig. 2c ), suggesting that the oestrogen-biosynthetic ability of ASCs is not sensitive to dimensionality. 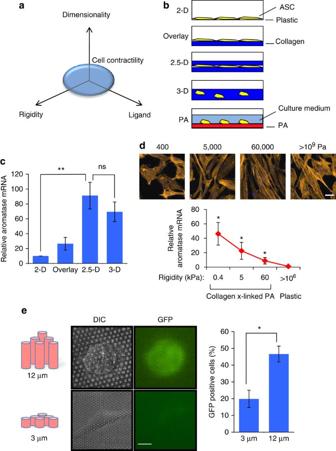Figure 2: Matrix compliance stimulates aromatase expression in ASCs. (a) Schematic illustration of multiple biomechanical parameters of ECM. (b) Diagram of various culture systems. (c) Aromatase expression is not responsive to dimensionality. NS, not significant. (d) Matrix compliance induces aromatase transcription. Stress fibres are detected by phalloidin staining (top). Scale bar, 50 μm. Aromatase mRNA expression is measured by RT–PCR. (e) High compliance as engineered in a micropost system confers stronger aromatase transcription. Left: differential interference contrast (DIC) and fluorescent images of I.3/PII-GFP reporter-containing ASCs, cultured on tall (12 μm) or short (3 μm) microposts. Right: quantification of GFP+ cells. Scale bar, 10 μm. NS, not significant,*P<0.05, **P<0.01, Student’st-test. Data represent mean±s.e.m. of three independent experiments. Figure 2: Matrix compliance stimulates aromatase expression in ASCs. ( a ) Schematic illustration of multiple biomechanical parameters of ECM. ( b ) Diagram of various culture systems. ( c ) Aromatase expression is not responsive to dimensionality. NS, not significant. ( d ) Matrix compliance induces aromatase transcription. Stress fibres are detected by phalloidin staining (top). Scale bar, 50 μm. Aromatase mRNA expression is measured by RT–PCR. ( e ) High compliance as engineered in a micropost system confers stronger aromatase transcription. Left: differential interference contrast (DIC) and fluorescent images of I.3/PII-GFP reporter-containing ASCs, cultured on tall (12 μm) or short (3 μm) microposts. Right: quantification of GFP+ cells. Scale bar, 10 μm. NS, not significant, *P <0.05, ** P <0.01, Student’s t -test. Data represent mean±s.e.m. of three independent experiments. Full size image Next, we used a widely adopted polyacrylamide (PA) gel system ( Fig. 2b ) to assess the impact of matrix rigidity/compliance on aromatase expression. At a constant concentration of crosslinked collagen, rigidity of the underlying PA gel can be readily manipulated by altering the ratio of acrylamide and bis-acrylamide [25] . We chose a range of bis-acrylamide ratios with elastic moduli ranging from one near that of adipose tissue (150–200 Pa) [26] , [27] to one approximating neoplastic tissue (5,000 Pa) and beyond. As expected, actin stress fibres detected by phalloidin staining were prominent in ASCs cultured on plastic and on stiff, but not soft, PA gels (top panel in Fig. 2d ). Increasing matrix compliance (or decreasing rigidity) resulted in decreased actin stress fibre formation and, surprisingly, a marked induction in aromatase mRNA levels (graph in Fig. 2d ). To confirm that the matrix compliance-dependent stromal aromatase expression is not limited to PA gels [28] , we employed a recently developed micropost system in which different rigidities are achieved by varying micropost height ( Fig. 2e ) [29] . Using the aromatase I.3/PII-GFP reporter as the readout of aromatase transcription ( Fig. 1f ), we found that ASCs on the taller, thus more compliant, micropost substrate expressed more aromatase than ASCs cultured on the shorter, stiffer microposts ( Fig. 2e ). Collectively, these observations indicate that matrix compliance is an important biomechanical stimulus for stromal aromatase gene expression. Cell contractility is inhibitory for aromatase expression Cells respond to substratum rigidity by altering cytoskeletal dynamics and adopting a certain degree of cell contractility, which in turn can influence different cellular functions [30] . To determine whether cell contractility alone affects stromal aromatase expression, ASCs cultured under a constant substrate rigidity were treated with three pharmacological inhibitors that prevented actin polymerization. They were the Rho-associated protein kinase inhibitor Y-27632, non-muscle myosin II inhibitor Blebbistatin, and actin polymer (F-actin) inhibitor Latrunculin A ( Fig. 3a ). All three inhibitors decreased cell size and disrupted actin stress fibre formation to various degrees ( Fig. 3a ), which correlated with striking increases in aromatase expression ( Fig. 3a ; note the log scale). 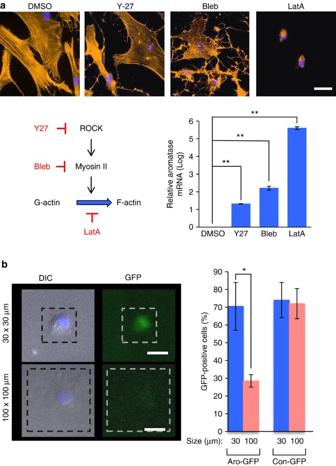Figure 3: Cell contractility is an inhibitory cue for stromal aromatase expression. (a) Effects of cytoskeleton-destabilizing agents on stromal aromatase transcription and stress fibre formation. Scale bar, 50 μm. Note the log scale for the relative aromatase mRNA levels. (b) Smaller cell size confers higher aromatase expression. Left, DIC and fluorescent micrographs of I.3/PII-GFP reporter-containing ASCs cultured on small (30 × 30 μm2) and large (100 × 100 μm2) micropatterned islands. Right: quantification of GFP-positive cells, containing either an aromatase I.3/PII-driven GFP (Aro-GFP) or a constitutively active promoter-driven GFP reporter (Con-GFP). *P<0.05, **P<0.01, Student’st-test. Data represent mean±s.e.m. of three independent experiments. Scale bar, 30 μm. Figure 3: Cell contractility is an inhibitory cue for stromal aromatase expression. ( a ) Effects of cytoskeleton-destabilizing agents on stromal aromatase transcription and stress fibre formation. Scale bar, 50 μm. Note the log scale for the relative aromatase mRNA levels. ( b ) Smaller cell size confers higher aromatase expression. Left, DIC and fluorescent micrographs of I.3/PII-GFP reporter-containing ASCs cultured on small (30 × 30 μm 2 ) and large (100 × 100 μm 2 ) micropatterned islands. Right: quantification of GFP-positive cells, containing either an aromatase I.3/PII-driven GFP (Aro-GFP) or a constitutively active promoter-driven GFP reporter (Con-GFP). * P <0.05, ** P <0.01, Student’s t -test. Data represent mean±s.e.m. of three independent experiments. Scale bar, 30 μm. Full size image We then employed a micropatterning approach [31] to assess a direct impact of cell size on aromatase expression without pharmacologically inhibiting the actin-polymerizing apparatus. When seeded on micropatterned islands of different sizes, individual ASCs with the integrated aromatase I.3/PII-GFP reporter adapted themselves to the confined area of a given island ( Supplementary Fig. S2a ). To avoid any confounding effect of cell–cell interactions, only islands seeded with single cells were included in our analysis. As expected, cells on smaller islands (30 × 30 μm 2 ) contained less stress fibre formation (thus low contractility) when compared with their counterparts on larger islands (100 × 100 μm 2 ; Supplementary Fig. S2b ). On the other hand, space-confined cells gave rise to more GFP+ cells than the larger ones ( Fig. 3b ). The cell size/contractility-dependent GFP expression appears to be specific to the I.3/PII aromatase promoter, as a GFP reporter driven by a control promoter (EF1-α) was not significantly affected by the same geometrical change ( Fig. 3b ). These experiments strongly suggest that high cell contractility is an inhibitory cue for stromal aromatase expression. DDR1 and integrin β1 mediate the biomechanical cues Given the mutually antagonizing effects of matrix compliance and cell contractility on stromal aromatase transcription, we reasoned that collagen in the 3-D system exerted two disparate actions on ASCs. When compared with highly rigid 2-D plastic substrata, collagen provides a relatively compliant substratum and therefore sustains high aromatase transcription. At the same time, collagen–cell interactions promote cell contractility, which would partially offset compliance-stimulated aromatase expression in the 3-D system. To separate these two antagonistic functions of collagen, we reduced or completely omitted collagen that was otherwise crosslinked to ‘activated’ PA for improving cell adhesion. We rationalized that, when its stimulatory role as a compliant substratum was substituted by PA, collagen would be entirely inhibitory for aromatase transcription. As shown in Fig. 4a , ASCs were still able to attach to the PA surface even in the absence of exogenous collagen. This was likely due to the fact that ASCs under compliant conditions expressed elevated levels of endogenous ECM proteins, as revealed by immunofluorescent staining ( Supplementary Fig. S3a ) and gene expression profiling ( Supplementary Table S1 ). As predicted, reduction or omission of exogenous collagen from the PA system resulted in further increases in aromatase expression ( Fig. 4a ). The inhibitory activity of collagen was not simply due to enhanced cell adhesion, as poly- L -lysine, a commonly used attachment reagent in cell culture, had no effects on aromatase mRNA levels on PA gels ( Supplementary Fig. S3b ). It is also notable that, in contrast to collagen-crosslinked PA, poly- L -lysine-coated PA did not induce stress fibre formation or cell spreading ( Supplementary Fig. S3c ). Thus, the ligand function of collagen in promoting stress fibre formation most likely accounts for attenuated aromatase transcription in the presence of crosslinked collagen. 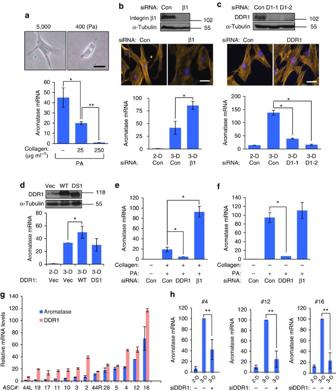Figure 4: DDR1 and β1 integrin mediate the effects of compliance and contractility, respectively. (a) Decreasing amounts of crosslinked collagen result in more aromatase mRNA in the PA (400 Pa) system. The DIC images show that ASCs are attached to PA without crosslinked exogenous collagen. Scale bar, 50 μm. (b,c) Effect of integrin β1 (b) or DDR1 (c) knockdown on stress fibre formation in 2-D and aromatase transcription in 3-D. The immunoblots indicate the knockdown efficiency. Scale bar, 50 μm. (d) Effects of WT and mutant (DS1) DDR1 on aromatase transcription. (e) Effects of DDR1 and integrin β1 knockdown on aromatase transcription in ASCs cultured on PA gels (400 Pa) with crosslinked collagen (150 μg ml−1). (f) Effects of DDR1 and integrin β1 knockdown on aromatase transcription in the PA system (400 Pa) without crosslinked collagen. (g) Correlation between DDR1 and aromatase abundance in primary ASCs from various donors. (h) DDR1 knockdown in the top three ASC samples in (g) results in reduced aromatase mRNA levels. *P<0.05, **P<0.01, Student’st-test. Data represent mean±s.e.m. of three independent experiments. Figure 4: DDR1 and β1 integrin mediate the effects of compliance and contractility, respectively. ( a ) Decreasing amounts of crosslinked collagen result in more aromatase mRNA in the PA (400 Pa) system. The DIC images show that ASCs are attached to PA without crosslinked exogenous collagen. Scale bar, 50 μm. ( b , c ) Effect of integrin β1 ( b ) or DDR1 ( c ) knockdown on stress fibre formation in 2-D and aromatase transcription in 3-D. The immunoblots indicate the knockdown efficiency. Scale bar, 50 μm. ( d ) Effects of WT and mutant (DS1) DDR1 on aromatase transcription. ( e ) Effects of DDR1 and integrin β1 knockdown on aromatase transcription in ASCs cultured on PA gels (400 Pa) with crosslinked collagen (150 μg ml −1 ). ( f ) Effects of DDR1 and integrin β1 knockdown on aromatase transcription in the PA system (400 Pa) without crosslinked collagen. ( g ) Correlation between DDR1 and aromatase abundance in primary ASCs from various donors. ( h ) DDR1 knockdown in the top three ASC samples in ( g ) results in reduced aromatase mRNA levels. * P <0.05, ** P <0.01, Student’s t -test. Data represent mean±s.e.m. of three independent experiments. Full size image Type 1 collagen interacts with heterodimeric integrin receptors formed between the β1 subunit and one of several α subunits [32] . In addition, discoidin domain receptors 1 and 2 (DDR1 and DDR2) serve as non-integrin receptors for collagen [32] . We therefore asked whether these known collagen receptors mediated the dual effects of collagen on aromatase transcription. Knockdown of β1 integrin significantly reduced stress fibres ( Fig. 4b ) and further enhanced high aromatase mRNA levels in the 3-D system ( Fig. 4b ). In support, knockdown of downstream signalling molecules in the integrin-initiated pathway (FAK, Rac1 and RhoA) also led to augmented aromatase transcription ( Supplementary Fig. S4a–c ). This result suggests that β1 integrin is important for collagen-induced stress fibre formation and the ensuing inhibition of aromatase transcription. In contrast, cells with DDR1 knockdown still had intact stress fibre formation ( Fig. 4c ), indicating that DDR1 is not the primary collagen receptor in ASCs. However, DDR1 knockdown by two independent small interfering RNA (siRNA) oligos completely abolished 3-D-induced aromatase transcription ( Fig. 4c ). In addition, ectopic expression of wild-type (WT) DDR1, but not a mutant devoid of the discoidin (DS) domain [33] , further enhanced 3-D-stimulated aromatase mRNA levels ( Fig. 4d ). Knockdown of neither α2 integrin nor DDR2 resulted in any appreciable changes in aromatase mRNA levels ( Supplementary Fig. S4d-e ). Finally, when β1 integrin was depleted from ASCs, 3-D-stimulated aromatase transcription was still dependent on DDR1 ( Supplementary Fig. S4f ). Taken together, these results indicate that DDR1 and β1 integrin act independently to mediate the two opposite effects of collagen on stromal aromatase transcription under the 3-D conditions. To further elucidate the distinct roles of DDR1 and β1 integrin in mediating various effects of collagen on aromatase transcription, we conducted similar knockdown experiments in the PA system, with ( Fig. 4e ) or without exogenous collagen ( Fig. 4f ). DDR1 knockdown significantly reduced aromatase mRNA levels regardless of the presence of exogenous collagen ( Fig. 4e ). In contrast, knockdown of β1 integrin only enhanced aromatase expression when collagen was included in the system ( Fig. 4e ). No effects of β1 knockdown were observed in the absence of collagen ( Fig. 4f ). These findings clearly indicate that DDR1 and β1 integrin mediate the opposite effects of collagen on aromatase transcription. Although DDR1 is not a major collagen receptor in ASCs, it might still require the ligand interaction of collagen to mediate compliance-stimulated aromatase transcription. However, we do not favour this possibility as DDR1 supports aromatase transcription in the PA system even in the absence of any exogenous collagen ( Fig. 4f ). Furthermore, Matrigel or a synthetic hydrogel (PuraMatrix) stimulated aromatase transcription to similar degrees as the type 1 collagen 3-D gels ( Supplementary Fig. S4g–h ). Lastly, a synthetic triple-helical collagen peptide known to specifically bind to DDR1 [34] , [35] did not stimulate aromatase transcription in ASCs cultured on plastic ( Supplementary Fig. S4i ). These results suggest that the ligand–receptor interaction is not involved in DDR1-mediated aromatase transcription. To further verify the functional relationship between DDR1 and aromatase expression, we analysed the mRNA levels of both genes in a cohort of primary ASCs isolated from cancer-free individuals who underwent reduction mammoplasty. As shown in Fig. 4g , there is a remarkable correlation between mRNA expression of DDR1 and aromatase (Pearson’s correlation coefficient: 0.95; P <0.00001). Importantly, DDR1 knockdown in three different samples with high DDR1/aromatase expression substantially reduced aromatase mRNA ( Fig. 4h ), thus demonstrating the causality between these two genes. JNK1 and phospho-JunB mediate the cue of matrix compliance DDR1 is known to activate several members of the mitogen-activated kinase family including c-Jun N-terminal kinase (JNKs) and p38 kinases [36] . ASCs embedded in the collagen-based 3-D microenvironment exhibited enhanced phosphorylation of JNK, but not p38 ( Fig. 5a ). Importantly, the 3-D-induced JNK phosphorylation was obliterated upon DDR1 knockdown ( Fig. 5b ), thus placing JNK activation downstream of DDR1. Several lines of evidence further confirmed that activated JNK is functionally involved in 3-D-induced aromatase transcription. First, pharmacological inhibition of JNK (AS-601245), but not p38 (SB-203580), eliminated aromatase transcription ( Fig. 5c ) that was driven by the I.3 and PII promoters ( Fig. 5d ). A similar inhibitory effect of the JNK inhibitor was also observed in the compliant PA system ( Fig. 5e ). In addition, siRNA knockdown of JNK1 significantly reduced aromatase mRNA level in the 3-D system ( Fig. 5f ). Lastly, ectopic expression of WT, but not a catalytically dead mutant, JNK1 stimulated aromatase transcription ( Fig. 5g ). 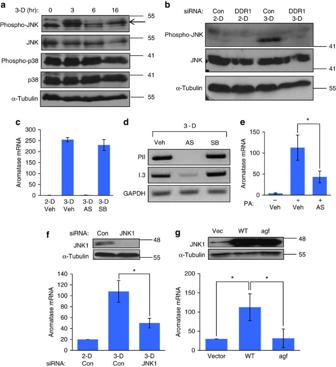Figure 5: JNK signaling pathway transduces the biomechanical signals to aromatase transcription. (a) JNK and p38 phosphorylation in 3-D ASCs. The arrow points to the position of phospho-JNK. (b) Phosphorylated and total JNK in control and DDR1 knockdown ASCs. (c) Aromatase mRNA in 3-D ASCs in the presence and absence of AS-601245 (AS; JNK inhibitor) and SB-203580 (SB; p38 inhibitor). (d) Effects of AS and SB on promoter-specific aromatase transcripts in 3-D ASCs. (e) Effect of AS on aromatase transcription in ASCs cultured in the compliant PA system (400 Pa) without crosslinked collagen. (f) ECM-stimulated aromatase mRNA in control and JNK-1 depleted ASCs. (g) Effects of WT and mutant (agf) JNK-1 on aromatase transcription. *P<0.05, Student’st-test. Data represent mean±s.e.m. of three independent experiments. Figure 5: JNK signaling pathway transduces the biomechanical signals to aromatase transcription. ( a ) JNK and p38 phosphorylation in 3-D ASCs. The arrow points to the position of phospho-JNK. ( b ) Phosphorylated and total JNK in control and DDR1 knockdown ASCs. ( c ) Aromatase mRNA in 3-D ASCs in the presence and absence of AS-601245 (AS; JNK inhibitor) and SB-203580 (SB; p38 inhibitor). ( d ) Effects of AS and SB on promoter-specific aromatase transcripts in 3-D ASCs. ( e ) Effect of AS on aromatase transcription in ASCs cultured in the compliant PA system (400 Pa) without crosslinked collagen. ( f ) ECM-stimulated aromatase mRNA in control and JNK-1 depleted ASCs. ( g ) Effects of WT and mutant (agf) JNK-1 on aromatase transcription. * P <0.05, Student’s t -test. Data represent mean±s.e.m. of three independent experiments. Full size image Jun proteins are the known targets of JNK kinases. Knockdown of JunB, but not c-Jun, significantly reduced ECM-stimulated aromatase expression ( Fig. 6a ) through the I.3/PII promoters ( Fig. 6b ). JunB knockdown also reduced the aromatase transcription in the compliant PA system ( Fig. 6c ). In a reciprocal approach, ectopic expression of WT JunB stimulated aromatase expression ( Fig. 6d ). Importantly, a JunB mutant (ala) that lacks two previously identified JNK-phosphorylation sites (Threonine 102 and 104) [37] failed to activate aromatase transcription ( Fig. 6d ). Using chromatin immunoprecipitation (ChIP), we found that JunB binding to the I.3/PII promoter was enhanced when ASCs were cultured in the 3-D microenvironment ( Fig. 6e ). Interestingly, mutation of the JNK-phosphorylation sites in JunB resulted in less efficient chromatin occupancy ( Fig. 6e ), suggesting that enhanced JunB chromatin binding upon JNK phosphorylation contributes to the elevated aromatase transcription from the I.3/PII promoters. 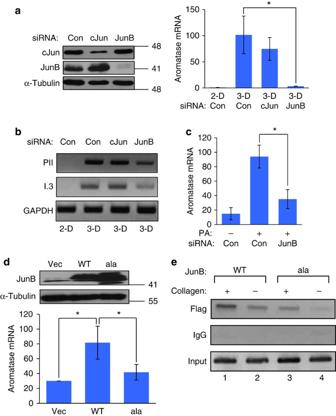Figure 6: JNK-mediated JunB phosphorylation stimulates aromatase transcription in ASCs. (a) Effects of c-Jun and JunB knockdowns on ECM-induced aromatase mRNA expression. (b) Effects of c-Jun and JunB depletion on ECM-stimulated transcription from the proximal aromatase promoters (PII and 1.3). (c) JunB knockdown reduces aromatase transcription in the compliant PA system (400 Pa). (d) Effects of ectopic expression of WT and mutant (ala) JunB proteins on aromatase mRNA in collagen-embedded 3-D ASCs. (e) ChIP detects differential occupancy of WT and mutant Flag-JunB at the proximal aromatase promoters. *P<0.05, Student’st-test. Data represent mean±s.e.m. of three independent experiments. Figure 6: JNK-mediated JunB phosphorylation stimulates aromatase transcription in ASCs. ( a ) Effects of c-Jun and JunB knockdowns on ECM-induced aromatase mRNA expression. ( b ) Effects of c-Jun and JunB depletion on ECM-stimulated transcription from the proximal aromatase promoters (PII and 1.3). ( c ) JunB knockdown reduces aromatase transcription in the compliant PA system (400 Pa). ( d ) Effects of ectopic expression of WT and mutant (ala) JunB proteins on aromatase mRNA in collagen-embedded 3-D ASCs. ( e ) ChIP detects differential occupancy of WT and mutant Flag-JunB at the proximal aromatase promoters. * P <0.05, Student’s t -test. Data represent mean±s.e.m. of three independent experiments. Full size image Consequence of compliance-stimulated oestrogen production To ascertain the functional consequence of matrix compliance-induced aromatase expression in ASCs, we assessed the impact of stromal oestrogen production on oestrogen-dependent transcription in ER+ breast cancer cell lines ZR75-1 and MCF-7. As illustrated in Fig. 7a , when ASCs were cultured under the 3-D condition in the presence of the aromatase substrate testosterone, elevated aromatase expression led to more robust oestrogen synthesis and increased secretion of oestrogen into the culture medium. As a functional readout, ASC-conditioned medium was then added to ER+ breast cancer cells that were deprived of oestrogens, and oestrogen-dependent gene transcription in these cancer cells was measured. As expected, transcription of aromatase in ASCs was significantly elevated in the 3-D conditions, with and without testosterone ( Fig. 7b ). When medium conditioned by 3-D ASCs was added to ZR75-1 breast cancer cells, mRNA levels of pS2, a prototypical oestrogen-responsive gene, was substantially elevated in the cancer cells ( Fig. 7c ). Importantly, the stimulatory effect of the 3-D cultured ASC-conditioned medium depended on addition of the aromatase substrate testosterone to ASCs ( Fig. 7c ). In contrast, no testosterone-dependent effects were observed in the conditioned medium that was collected from ASCs cultured in 2-D conditions ( Fig. 7c ), demonstrating that testosterone only becomes stimulatory when sufficient stromal aromatase is expressed in the 3-D ASC culture. Furthermore, when the AI letrozole was added to 3-D ASC cultures, it completely eliminated the effect of ASC-conditioned medium on pS2 transcription ( Fig. 7d ). A similar observation was made for a different oestrogen-responsive gene PDZK1 ( Supplementary Fig. S5a-b ) and in a different ER+ breast cancer cell line MCF-7 ( Supplementary Fig. S5c-d ). Thus, both the enzyme and substrate in oestrogen synthesis are required for the effect of 3-D ASC-conditioned medium on oestrogen-responsive transcription in ER+ breast cancer cells. Lastly, DDR1 knockdown in 3-D cultured ASCs significantly reduced the effect of the corresponding conditioned medium on oestrogen-dependent transcription in breast cancer cells ( Fig. 7e ), further supporting the notion that DDR1-mediated stromal aromatase expression and oestrogen production ultimately result in activation of oestrogen-dependent transcription in breast cancer cells. 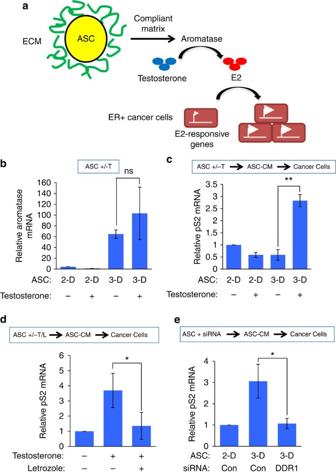Figure 7: ECM-elevated stromal oestrogens stimulate oestrogen-dependent transcription in ER+ breast cancer cells. (a) Illustration of the experiments with the ASC-conditioned medium. Arrows in ER+ cancer cells denote transcription of oestrogen (E2)-dependent genes. (b) Aromatase mRNA expression in the 2-D or 3-D ASCs, with or without testosterone (T). (c) When 3-D ASCs are cultured in the presence of testosterone (T), the resulting ASC-conditioned medium (CM) stimulates oestrogen-dependent transcription of pS2 in ER+ breast cancer cells ZR75-1. (d) Effect of ASC-conditioned medium on oestrogen-dependent transcription in ZR75-1 cells is abolished by addition of AI letrozole (L) to the 3-D ASCs. (e) The effect of 3-D ASCs on oestrogen-dependent transcription of pS2 in ZR75-1 is abrogated when stromal DDR1 is knocked down in ASCs. NS, not significant, *P<0.05, **P<0.01, Student’st-test. Data represent mean±s.e.m. of three independent experiments. Figure 7: ECM-elevated stromal oestrogens stimulate oestrogen-dependent transcription in ER+ breast cancer cells. ( a ) Illustration of the experiments with the ASC-conditioned medium. Arrows in ER+ cancer cells denote transcription of oestrogen (E2)-dependent genes. ( b ) Aromatase mRNA expression in the 2-D or 3-D ASCs, with or without testosterone (T). ( c ) When 3-D ASCs are cultured in the presence of testosterone (T), the resulting ASC-conditioned medium (CM) stimulates oestrogen-dependent transcription of pS2 in ER+ breast cancer cells ZR75-1. ( d ) Effect of ASC-conditioned medium on oestrogen-dependent transcription in ZR75-1 cells is abolished by addition of AI letrozole (L) to the 3-D ASCs. ( e ) The effect of 3-D ASCs on oestrogen-dependent transcription of pS2 in ZR75-1 is abrogated when stromal DDR1 is knocked down in ASCs. NS, not significant, * P <0.05, ** P <0.01, Student’s t -test. Data represent mean±s.e.m. of three independent experiments. Full size image To examine the impact of stromal oestrogen production on the growth of ER+ breast cancer cells, we co-cultured ASCs with the ER+ breast cancer cells under 3-D conditions ( Fig. 8a ). As in the transcription studies described above, the cancer cells were starved in oestrogen-free medium before the co-culture. To distinguish the stromal and cancer cells in the co-culture system, ZR75-1 cells were integrated with a constitutively active GFP expression vector. The presence of ASCs in the 3-D system clearly stimulated proliferation of the cancer cells, as evidenced by the increased number of GFP+ cells ( Fig. 8a ). Importantly, this stimulatory effect of 3-D co-cultured ASCs was abolished by either the omission of the aromatase substrate testosterone or the addition of the AI letrozole ( Fig. 8b ). Testosterone alone did not affect the growth of the cancer cells per se ( Supplementary Fig. S6a ). To directly assess the stromal effect on DNA synthesis in the breast cancer cells, we applied either 2-D or 3-D ASC-conditioned medium to oestrogen-deprived ZR75-1 cells and subsequently pulse-labeled the cancer cells with bromo-deoxyuridine (BrdU). 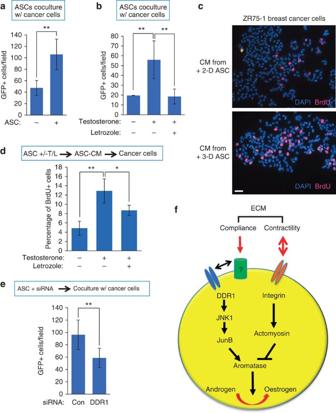Figure 8: ECM-elevated stromal oestrogen stimulates oestrogen-dependent growth of ER+ breast cancer cells. (a) ASCs stimulate growth of GFP+ breast cancer cells ZR75-1 in the 3-D co-culture system in the presence of the aromatase substrate testosterone. ZR75-1 cells, which are distinguished from ASCs by GFP expression, are starved in oestrogen-free medium before the co-culture. GFP+ cells in the co-culture system are scored. (b) 3-D ASC-mediated stimulation of ZR75-1 cancer cell growth depends on the presence of testosterone, and is abolished by letrozole. (c) ZR75-1 cells are pulse-labeled with BrdU, following exposure to 2-D or 3-D ASC-conditioned medium. Scale bar, 50 μm. (d) Quantitation of BrdU incorporation in ZR75-1 cells following exposure to ASC-conditioned medium. (e) DDR1 knockdown in 3-D ASCs reduces their ability to promote GFP+ ZR75-1 cancer cell growth. (f) An illustration of the DDR1- and β1 integrin-dependent pathways that antagonistically control aromatase transcription in the 3-D microenvironment. The question mark denotes the putative sensor for matrix compliance. The double arrow indicates reciprocity of the matrix–cell interaction in determining cell contractility. *P<0.05, **P<0.01, Student’st-test. Data represent mean±s.e.m. of three independent experiments. As shown in Figure 8c , conditioned medium from 3-D ASCs gave rise to a much greater number of BrdU+ cancer cells than medium conditioned by 2-D ASCs in the presence of testosterone. Again, the stimulatory effect of the 3-D ASC was dependent on testosterone and sensitive to letrozole ( Fig. 8d ). A similar effect of 3-D ASCs was also observed with MCF-7 breast cancer cells ( Supplementary Fig. S6b-c ). Lastly, knockdown of stromal DDR1 significantly reduced the ASC-mediated stimulation of tumour cell growth ( Fig. 8e ). Taken together, these experiments substantiate the notion that ECM-stimulated oestrogen output of ASCs constitutes a functionally important component of the hormonal communication between stromal cells and cancer cells in the tumour microenvironment. Figure 8: ECM-elevated stromal oestrogen stimulates oestrogen-dependent growth of ER+ breast cancer cells. ( a ) ASCs stimulate growth of GFP+ breast cancer cells ZR75-1 in the 3-D co-culture system in the presence of the aromatase substrate testosterone. ZR75-1 cells, which are distinguished from ASCs by GFP expression, are starved in oestrogen-free medium before the co-culture. GFP+ cells in the co-culture system are scored. ( b ) 3-D ASC-mediated stimulation of ZR75-1 cancer cell growth depends on the presence of testosterone, and is abolished by letrozole. ( c ) ZR75-1 cells are pulse-labeled with BrdU, following exposure to 2-D or 3-D ASC-conditioned medium. Scale bar, 50 μm. ( d ) Quantitation of BrdU incorporation in ZR75-1 cells following exposure to ASC-conditioned medium. ( e ) DDR1 knockdown in 3-D ASCs reduces their ability to promote GFP+ ZR75-1 cancer cell growth. ( f ) An illustration of the DDR1- and β1 integrin-dependent pathways that antagonistically control aromatase transcription in the 3-D microenvironment. The question mark denotes the putative sensor for matrix compliance. The double arrow indicates reciprocity of the matrix–cell interaction in determining cell contractility. * P <0.05, ** P <0.01, Student’s t -test. Data represent mean±s.e.m. of three independent experiments. Full size image The tumour microenvironment consists of three critical components, namely, tumour cells, stromal cells and ECM. Our study elucidates a previously unrecognized mechanism that links the biomechanical signals from ECM with endocrine output of adipose tissue-derived cells and consequently, the corresponding stromal impact on proliferation of ER+ breast tumour cells. Dissection of various ECM parameters allows us to uncover two distinct and diametrically opposing pathways that regulate stromal aromatase transcription and oestrogen production ( Fig. 8f ). On the one hand, matrix compliance triggers a DDR1-dependent signalling pathway that ultimately leads to activation of two breast cancer-associated aromatase promoters. On the other hand, a β1 integrin-dependent cytoskeleton network inhibits aromatase transcription at least in part through collagen–integrin interaction and stress fibre formation. An antagonistic interaction between DDR1 and β1 integrin was previously reported in migration of epithelial cells [38] , [39] . We propose that, in the stromal compartment of the breast, ASCs dynamically monitor biophysical properties of the ECM and integrate this biomechanical input to control endocrine and paracrine output. Our study identifies several key players, including DDR1, JNK1 and JunB, that mediate the matrix compliance-stimulated aromatase transcription. How exactly the mechanical cue is sensed, however, remains to be elucidated. Our data suggest that the ligand–receptor interaction between collagen and DDR1 is unlikely to be involved in the DDR1-mediated aromatase transcription. It is not clear whether DDR1 is involved in the initial sensing of matrix compliance or acts downstream of a putative mechanosensor in ASCs to transduce the mechanical signal ( Fig. 8f ). Distinguishing these two possibilities has been critical yet often challenging in studies of a number of other candidate mechanotransducers [40] , [41] . In this regard, it is worth noting that DDR1 knockout mice exhibit inner ear defects and hearing loss [42] , a sensory function that is intimately linked with mechanotransduction. Elevated circulating and local oestrogen levels are considered to be the primary contributing factor for obesity-associated breast cancer risk among postmenopausal women [6] . Although the overall increase in tissue mass clearly augments the total adipose oestrogen output in obese individuals, changes in the local extracellular milieu can also alter the oestrogen-synthetic capability of individual ASCs. For example, it is known that inflammatory factors such as prostaglandin E 2 and cytokines can stimulate aromatase expression by activating the I.3/PII promoters [13] , [14] , [16] . Likewise, it is conceivable that increased number and size of fat-laden adipocytes in adipose tissue of obese individuals could result in less tissue density and higher compliance, which may in turn potentiate robust aromatase transcription in neighbouring ASCs. Together with the biochemical cues from soluble factors, the biomechanical signals defined here could significantly promote obesity-related diseases by enhancing the oestrogen output of adipose tissue. We further predict that targeting the DDR1-dependent pathway may effectively reduce stromal oestrogen production and therefore offer therapeutic value. Recent studies of breast cancer cells indicate that increased matrix stiffening promotes tumour progression by elevating integrin signalling and focal adhesions [4] , [26] , [43] , [44] , [45] . In this regard, it seems counter-intuitive that more compliant ECM microenvironment is conducive to stromal oestrogen production and growth of ER+ breast tumour cells. Our finding illustrates the complexities of mechanical phenotype with regards to tumours of different ER status, tumour versus stromal cells, and proximity of fatty stroma to tumour cells. In addition, recent reports indicate that compliant ECM selects for tumour cells with enhanced tumorigenic capacity [46] , [47] . Therefore, ECM rigidity may have distinct, and even opposite, effects on different cell populations within the same tumour microenvironment. Although the current study primarily focused on the stromal oestrogen-mediated effects, ASCs are known to exert oestrogen-independent paracrine and endocrine actions [48] , [49] . Indeed, gene expression profiling indicates that a large number of ECM-encoding genes were induced in ASCs embedded in the 3-D microenvironment ( Supplementary Table S1 ). Moreover, ECM-stimulated genes in 3-D ASCs overlap significantly ( P <2 × 10 −12 ) with a previously published signature of stromal genes associated with invasive ductal carcinoma [50] . Interestingly, the DDR1 gene itself was highly induced in both 3-D culture and cancer-associated patient stroma. Of note, a recent study shows that tumour-secreted soluble factors can alter behaviours of ASCs and mechanical properties of the tumour microenvironment [51] . Therefore, mechanical phenotype as dictated by heterotypic interactions of different components of the tissue microenvironment may have a broad impact on the endocrine/paracrine functions of stromal cells beyond its oestrogen output. Aside from its association with pathogenesis, tissue-selective aromatase expression and local oestrogen production have key roles in supporting normal organ functions in a variety of tissues, including bone, brain and the cardiovascular system [52] , [53] . Given the diverse range of mechanical properties of these tissues (for example, from compliant brain tissue to the extremely rigid bone), it will be of interest to determine whether a given tissue-specific aromatase promoter is more responsive to a particular matrix rigidity corresponding to that of its native tissue microenvironment. It is also possible that changes in the mechanical properties could profoundly alter local oestrogen production and thus oestrogen-dependent tissue functions. Cell culture and related reagents Primary ASCs from breast or abdominal adipose tissue were procured from women undergoing elective surgical procedures and cultured using methods previously published and approved by the Institutional Human Investigation Committees [54] . MCF-7 and ZR75-1 cells were purchased from American Tissue Culture Center (ATCC). Latrunculin A, Blebbistatin, Y-27632, AS-601245, and SB-203580 were purchased from EMD Biosciences (USA). DDR1-binding and control peptides were described previously [34] , [35] and generously provided by Dr Richard Farndale’s laboratory (University of Cambridge). siRNA transfections Knockdown by siRNA oligonucleotides were conducted as previously described [55] , using Lipofectamine reagent RNAiMAX (Invitrogen). Control (D-001810-10), siDDR1-1 (D-00311-09) and siDDR1-2 (D-00311-10), siDDR2 (M-003112-04), siIntegrin α2 (M-004566-02), siIntegrin β1 (M-004506-00), siFAK (M-003164-02), siRhoA (M-003860-00), sicJun (M-003268-02), siJunB (M-003269-01) and siRac1(M-003560-06) were purchased from Dharmacon, Inc. (USA). siJNK-1 (SIHK 1219/1220/1221) were purchased from Sigma-Aldrich Inc. (USA). 3-D culture To culture ASCs in collagen, bovine type I collagen in acetic acid (BD Biosciences) was first neutralized by adding 10 × PBS (1/10 vol.) and 0.1 M NaOH (1/10 vol.) to reach pH 7.5. Desired number of cells were suspended in culture medium and mixed with neutralized collagen at 1:1 ratio (V/V) to reach a final concentration of 1.2 mg ml −1 and an approximate rigidity of 200 Pa [26] , [27] , which is close to the stiffness in normal breast tissue [27] , [28] . Cell–matrix mixtures were placed in tissue culture plates and were incubated for 20–30 min at 37 °C. Cell culture medium was then added carefully on top of the cultures, and cells were cultured for an additional 16 h. To harvest cells for RNA and protein analysis, the collagen-embedded cultures were digested with collagenase (Sigma) for 10 min at 37 °C. Digested products were spun down at 3,000 r.p.m. for 5 min at 4 °C and washed with PBS. The cell pellets were subjected to standard protein or RNA extraction. For the experiments shown in Supplementary Fig. S4g–h , 2 × 10 5 ASCs were mixed with Matrigel (Sigma, USA) (9.8 mg ml −1 ) or PuraMatrix (BD Biosciences, USA) in 1:1 ratio and were cultured overnight in 24-well tissue culture plates. Cells were harvested using cell-recovering solution (BD Biosciences, USA). Micropatterning Micropatterned glass coverslips of variable sizes were prepared following the published protocol [56] . Micropatterned coverslips were coated with fibronectin (10 μg ml −1 ) for 1 h at room temperature. Coverslips were washed 3 times with PBS, and ASCs were seeded on each coverslip at a density of 5,000 cells per cm 2 (dish area). After 30 min of incubation at 37 °C, the nonattached cells were removed by gently aspirating the medium and additional medium was added to the plates. Micropost The elastomeric poly (dimethylsiloxane) micropost arrays were obtained from Dr Christopher S Chen (University of Pennsylvania, USA). They were prepared for cell attachment using micro-contact printing, attached on the mattek dishes and coated with fibronectin as previously described [29] . Trypsinized ASCs at a density of 5,000 cells per cm 2 (dish area) were seeded on the imprinted mattek dishes. PA gel culture PA gels with calibrated stiffness were prepared as described previously [57] . In brief, glass coverslips were coated with silane (Sigma). PA gels were prepared with variable rigidities by mixing different ratios of bis-acrylamide and acrylamide and sulfo-SANPAH (Sigma). The gels were photoactivated with ultraviolet. Unless otherwise specified, gels were crosslinked overnight with type I collagen (150 μg ml −1 ) and cells were seeded on top of the gels. 2-D collagen substratum For overlaying the ASCs on top of the collagen layer, cell culture plates were coated with type I collagen (1.2 mg ml −1 ) and incubated for 2 h at room temperature. ASCs were then seeded on top of the solidified gel. For 2.5-D experiments, type I collagen (final concentration of 1.2 mg ml −1 ) was added on top of above-mentioned overlaid ASCs, 4 h after the initial cell seeding. The sandwiched ASCs were cultured for additional 12 h. Co-culture To perform the conditioned-medium experiment, both tumour cells and ASCs were cultured for 3 days in phenol red-free medium with charcoal-stripped serum. For some experiments as indicated, ASCs were cultured along with vehicle (ethanol), testosterone (10 nM) or testosterone with letrozole (10 μM). ASC-conditioned medium was then added to GFP-integrated, ER+ ZR75-1 or MCF-7 (non-GFP) cells (4 × 10 4 per well of 24-well plate). ASC-conditioned medium on cancer cells was changed daily and the cancer cells were cultured for a total of 5 days. In the physical co-culture experiment, ASCs (10 5 per well) and ZR75-1 (4 × 10 4 per well) were mixed together and cultured for 5 days inside collagen in phenol red-free medium with charcoal-stripped serum. BrdU pulse-labeling ZR75-1 and MCF-7 breast cancer cells and ASCs were cultured in phenol red-free medium with charcoal-stripped serum. Whenever indicated, ASCs were also incubated with testosterone and letrozole. After 3 days of starvation, the cancer cells were exposed to ASC-conditioned medium for 44 h. BrdU (final concentration of 50 μM) were added to the medium and the cancer cells were cultured for additional 4 h before harvesting for immunofluorescence. Cells were fixed and permeabilized. DNA was denatured (2 N HCl), followed by overnight incubation with an anti-BrdU antibody. Fluorescence microscopy and confocal microscopy To stain and visualize the actin stress fibres in ASCs, phalloidin staining was performed using F-actin visualization kit from Cytoskeleton (USA). The micropatterned coverslips were mounted using Vectashield mounting media with DAPI. Rhodamine and GFP were imaged using a Nikon Eclipse Ni with the × 40/0.75 NA objective lens. Images were taken with a Nikon DS-QiMC Black and White camera and analysed with Nikon Elements-Basic Research software. Live-Cell GFP micropost images were taken using a × 10/0.45 NA objective lens on a Nikon Eclipse TE300. Images were captured using a Nikon 6006 camera and analysed using Nikon Elements-Advanced Research Software. Antibodies For western blotting, the following antibodies were purchased from Cell Signalling (USA): JNK (9252), phospho-JNK (9255), p38 (9212) and phospho-p38 (4511). The following antibodies were purchased from Santa Cruz Biotech: c-Jun (sc-45), JunB (sc-8051) and DDR1 (sc532). Uncropped western blot images are provided in Supplementary Fig. S7 . In addition, the following antibodies were used: anti-α-tubulin (CP06; Calbiochem), anti-aromatase (MCA 20775; Serotec), and anti-Flag (M8, Sigma-Aldrich), anti-BrdU (RPN20Ab; GE Healthcare Life Sciences), and anti-collagen (ab59435, Abcam). Expression vectors and plasmid construction Wild-type DDR-1 and mutant (DDR1-DS1) that lacks the discoidin domain (amino acids 31–185) were gifts from Dr Eric Sahai. Both cDNAs were subcloned into the lentivirus expression vector (CD520A-1) purchased from System Biosciences (USA). JNK-1 and its mutant (JNK-1 agf) were purchased from Addgene (USA) and were subcloned between Nde I and Pme I in the modified pWPI vector (Addegene). Two threonine residues at positions 102 and 104 of human JunB were mutated to alanine by site-directed mutagenesis. Both WT and mutant JunB were cloned into the modified pWPI vector, with the addition of Flag-tag at the 5′ end of the cDNAs. To generate the I.3/PII-driven GFP reporter construct, the EF1-α promoter of the pWPXLd (Addgene) vector was replaced with a 1-kb genomic DNA fragment upstream of the aromatase gene. Lentiviruses were generated and amplified in 293T cells by co-transfection with the above-mentioned constructs and packaging vectors pMD2.G and psPAX2 (Addgene). Quantitative and semi-quantitative RT–PCR Total RNA was isolated using TRIzol reagent (Invitrogen) according to the manufacturer’s instructions. RNA was reverse-transcribed using the ImPrompII kit (Promega). Real-time PCR was carried out using the fluorescent dye SYBR-Green and an ABI 7900 Real-Time PCR System (Applied Biosystems) (Primer sequences listed in Supplementary Table S2 ). Semi-quantitative PCRs to detect promoter-specific aromatase transcripts were performed using aromatase exon I-specific primers as described previously [58] . Aromatase activity assay Aromatase activity assay using the ASCs was performed following the previously described method [58] . Chromatin immunoprecipitation ChIP protocol was performed by following the method as described in our previous publication [59] . In short, ASCs were recovered from the 2-D or 3-D culture by digestion with collagenase (Sigma-Aldrich), and were crosslinked with 1% formaldehyde for 10 min, followed by termination with 125 mM glycine for 5 min. Statistics Data presented in each figure represents a mean value of three independent biological experiments. The mean values±s.e.m. and statistical analysis were calculated and plotted using Microsoft Excel program. The two-tailed independent Student t -test was used to compare the continuous variables between two groups. Difference for all tests were considered significant when P -value was lower than 0.05. Microarray and bioinformatics analysis Whole-genome gene expression analysis was performed using the whole-genome DASL HT Assay, an updated version of the original whole-genome DASL assay [60] . Gene ontology analysis was then performed using Genespring GX software on all upregulated genes with a fold change of two-fold and higher and a P -value<0.05. The microarray data have been deposited in the Gene Expression Omnibus (GSE44811). Breast cancer-associated stromal signature as published previously [50] were extracted from the dataset (accession number GSE9014), downloaded from the NCBI GEO website. The upregulated genes were identified with fold-changes >4 between tumour and normal samples and compared with the upregulated genes selected from this study. The statistical significance ( P -value) of the overlap was calculated using the Fisher’s exact test: where N is the total number of genes in the experiment; m,n is the selected upregulated gene and o is the overlap among those upregulated genes. C(n,k) is the bionomial coefficient. Accession codes: Microarray data have been deposited in the Gene Expression Omnibus under accession code GSE44811 . How to cite this article: Ghosh, S. et al . Regulation of adipose oestrogen output by mechanical stress. Nat. Commun. 4:1821 doi: 10.1038/ncomms2794 (2013).